Activation of the NLRP1b inflammasome independently of ASC-mediated caspase-1 autoproteolysis and speck formation Despite its clinical importance in infection and autoimmunity, the activation mechanisms of the NLRP1b inflammasome remain enigmatic. Here we show that deletion of the inflammasome adaptor ASC in BALB/c mice and in C57BL/6 macrophages expressing a functional NLRP1b prevents anthrax lethal toxin (LeTx)-induced caspase-1 autoproteolysis and speck formation. However, ASC −/− macrophages undergo normal LeTx-induced pyroptosis and secrete significant amounts of interleukin (IL)-1β. In contrast, ASC is critical for caspase-1 autoproteolysis and IL-1β secretion by the NLRC4, NLRP3 and AIM2 inflammasomes. Notably, LeTx-induced inflammasome activation is associated with caspase-1 ubiquitination, which is unaffected in ASC-deficient cells. In vivo , ASC-deficient mice challenged with LeTx produce significant levels of IL-1β, IL-18 and HMGB1 in circulation, although caspase-1 autoproteolysis is abolished. As a result, ASC −/− mice are sensitive to rapid LeTx-induced lethality. Together, these results demonstrate that ASC-driven caspase-1 autoprocessing and speck formation are dispensable for the activation of caspase-1 and the NLRP1b inflammasome. The cysteine protease caspase-1 plays a central role in proteolytically maturing and secreting the cytokines pro-interleukin (IL)-1β and IL-18, and in inducing a pro-inflammatory programmed cell death mode termed pyroptosis [1] . In addition to IL-1β’s role as a critical pyrogen, both IL-1β and IL-18 shape innate and adaptive immune responses through a multitude of mechanisms that ultimately lead to coordinated host responses against infectious agents. In addition, recent reports highlighted a key role for caspase-1-mediated pyroptosis in controlling in vivo replication and dispersion of microbial pathogens [2] . Consequently, deregulated caspase-1 activation contributes importantly to a wide spectrum of infectious, autoimmune and inflammatory diseases [3] . To avoid unwarranted and potentially destructive immune responses, caspase-1 activation in innate immune cells is regulated at several steps. Caspase-1 is produced as a catalytically latent monomeric zymogen that resides in the cytosol of naive myeloid cells [4] . The zymogen consists of an amino-terminal caspase recruitment domain (CARD) that is separated from the catalytic protease domain by a short linker peptide. In addition, a short linker segregates the large (p20) and small (p10) subunits of the caspase proteolytic domain [5] . Imperative to gaining proteolytic activity, procaspase-1 needs to be recruited into cytosolic multi-protein complexes termed inflammasomes [4] . Inflammasome complexes are assembled in a pathogen- or danger-associated molecular pattern (DAMP)-specific manner, and routinely distinguished based on the NOD-like receptor (NLR) or HIN200 pattern recognition receptor (PRR) facilitating caspase-1 autoactivation in the complex [1] . Genetic studies in mice have confirmed the existence of at least four distinct inflammasomes responding to a diversity of PAMPs and DAMPs. The AIM2 inflammasome is assembled and activates caspase-1 when DNA is detected in the cytosolic compartment of macrophages infected with the DNA viruses cytomegalovirus and vaccinia virus, or the facultative intracellular bacterial pathogen Francisella tularensis [6] , [7] . The NLRP3 inflammasome is required for caspase-1 activation and IL-1β/IL-18 secretion in response to a broad range of bacterial, viral and fungal pathogens, as well as medically relevant crystalline substances, and endogenous danger-associated molecular patterns that have been linked to the etiology of autoimmune and auto-inflammatory disorders [1] . The NLRC4 inflammasome responds to a more restricted set of bacterial components. This inflammasome was namely shown to be responsible for caspase-1 activation upon cytosolic detection of bacterial flagellin or the conserved PrgJ basal body of bacterial type III secretion systems expressed by facultative intracellular pathogens such as S. typhimurium , S. flexneri , P. aeruginosa , B. thailandensis , and L. pneumophila [1] . Finally, the NLRP1b inflammasome is critical for caspase-1 activation by anthrax lethal toxin (LeTx), a key virulence factor of Bacillus anthracis [8] . Inhalation and ingestion of endospores of this Gram-positive rod-shaped bacterium is often fatal as a result of severe haemorrhagic disease. The spores are believed to target macrophages for their replication and systemic dispersion into the bloodstream [9] . Morbidity and mortality associated with systemic anthrax infection are caused by the tripartite anthrax toxin. The protective antigen (PA) subunit of the toxin binds to cell surface receptors of target cells and allows cytosolic entry of the metalloprotease lethal factor (LF) and the adenylate cyclase edema factor (EF) subunits. The combination of PA and EF (edema toxin) induces edema, whereas the combined action of PA and LF (called lethal toxin; LeTx) is responsible for lethal shock in experimental animals [9] . The differential susceptibility of inbred mouse strains to LeTx-induced macrophage cell death and in vivo lethality was mapped to the gene encoding NLRP1b [8] . Cytosolic presence of LF triggers assembly of a caspase-1-activating inflammasome complex in macrophages with a functional NLRP1b allele [10] . Recent studies showed that NLRP1b autoprocessing within the Function to Find Domain (FIIND) is required for LeTx-induced NLRP1b inflammasome activation [11] . Nevertheless, little is known about the molecular determinants and the mechanistic requirements leading to NLRP1b inflammasome-mediated caspase-1 activation, IL-1β secretion and cell death in LeTx-intoxicated macrophages and in in vivo -challenged animals. Particularly, the role of the inflammasome adaptor ASC in NLRP1b inflammasome signalling is debated due to the lack of appropriate ASC-deficient mouse models. Some reports relying on ectopic expression of inflammasome components suggested ASC to be dispensable for NLRP1b inflammasome signalling [12] , [13] , while other reports implicated ASC in NLRP1b inflammasome signalling [14] . Thus, the physiological role of ASC in NLRP1b inflammasome signalling remains to be fully addressed. Here, we show in two genetic backgrounds that ASC is critical for NLRP1b inflammasome-mediated caspase-1 autoproteolysis and speck formation. Surprisingly, however, ASC is dispensable for LeTx-induced IL-1β secretion and pyroptotic cell death. Moreover, we find that activation of the NLRP1b inflammasome is associated with the ubiquitination of caspase-1, which requires NLRP1b and caspase-1 enzymatic activity, but not ASC. As in cultured macrophages, in vivo caspase-1 autoprocessing is blunted in splenocytes of ASC-deficient mice challenged with LeTx, while they produce significant levels of IL-1β and IL-18, and release the danger signal HMGB1 in circulation. Consequently, these mice succumb to LeTx intoxication with similar kinetics as ASC +/+ littermates. ASC is critical for NLRP1b-mediated caspase-1 autoproteolysis Recent reports showed that enzymatic activity of LeTx [10] and a functional NLRP1b allele [8] were critical for caspase-1 activation in intoxicated macrophages. In agreement, PA-mediated delivery of wild-type LF—but not the catalytically inactive LF E687C mutant—potently triggered caspase-1 processing in bone marrow-derived macrophages (BMDMs) of BALB/c mice ( Fig. 1a ). Unlike the BALB/c mouse strain, C57BL/6J macrophages express a dysfunctional NLRP1b allele, rendering them resistant to LeTx-induced caspase-1 activation [8] . Consequently, the combination of PA and LF failed to trigger caspase-1 processing ( Fig. 1a ) and membrane lysis in C57BL/6J macrophages ( Fig. 1b ). The bipartite inflammasome adaptor ASC plays a critical role in the NLRP3, AIM2 and NLRC4 inflammasomes [15] , [16] , [17] , [18] , but in-depth analysis of its role in NLRP1b inflammasome signalling was hampered by the LeTx-resistant phenotype of C57BL/6J mice. To characterize the role of ASC in NLRP1b inflammasome signalling, C57BL/6J (B6) mice transgenic for a functional NLRP1b allele transcribed from its endogenous promoter (referred to as B6 Nlrp1b+ mice) were bred to ASC-deficient mice. NLRP1b and ASC genotyping allowed segregation of B6 Nlrp1b− (further referred to as B6), B6 Nlrp1b+ , B6 Nlrp1b+ ASC +/− and B6 Nlrp1b+ ASC −/− littermates ( Supplementary Fig. 1a ), and RT–PCR analysis confirmed that transcripts levels of the functional NLRP1b allele in NLRP1b-transgenic BMDMs were comparable to endogenous NLRP1b mRNA levels in 129SVEV57 macrophages ( Supplementary Fig. 1b ). Finally, western blot analysis confirmed intermediate ASC expression levels in B6 Nlrp1b+ ASC +/− cells and absent expression in B6 Nlrp1b+ ASC −/− macrophages ( Supplementary Fig. 1c ). In agreement with published results [18] , [19] , ASC plays a critical role in caspase-1 autoproteolysis by the NLRP3 inflammasome because nigericin-induced caspase-1 autoprocessing into the p20 subunit was evident in LPS-primed B6 and B6 Nlrp1b+ macrophages, but not in ASC −/− and B6 Nlrp1b+ ASC −/− cells ( Fig. 1c ). Similarly, ASC was necessary for caspase-1 autoprocessing by respectively the AIM2 and NLRC4 inflammasomes because transfection of double-stranded DNA (dsDNA) and infection with Salmonella typhimurium ( S. typhimurium ) induced caspase-1 maturation in B6 and B6 Nlrp1b+ macrophages, but not in ASC-deficient cells ( Fig. 1d,e ). To determine the role of ASC in caspase-1 autoproteolysis upon engagement of the NLRP1b inflammasome, macrophages of different genotypes were exposed to LeTx (10 μg ml −1 PA and LF, respectively) for 3 h before cell lysates were analysed for caspase-1 autoproteolysis. Unlike in B6 macrophages, LeTx potently induced caspase-1 autoproteolysis in B6 Nlrp1b+ macrophages that were or were not prestimulated with LPS ( Fig. 1f ). LeTx-induced caspase-1 processing was significantly reduced in macrophages from heterozygous B6 Nlrp1b+ ASC +/− littermates, and abolished in B6 Nlrp1b+ ASC −/− macrophages ( Fig. 1f ), suggesting a critical role for ASC in LeTx-induced caspase-1 autoproteolysis. Also, when exposed to a low concentration of LeTx (500 ng ml −1 PA and 250 ng ml −1 LF, respectively), caspase-1 autoproteolysis was readily detectable in lysates of B6 Nlrp1b+ macrophages ( Fig. 1g ). In contrast, caspase-1 processing was markedly reduced in macrophages of B6 Nlrp1b+ ASC +/− littermates, and fully absent in cells from B6 Nlrp1b+ ASC −/− mice ( Fig. 1g ). Together, these results confirm that ASC is critical for caspase-1 autoproteolysis by the NLRC4, NLRP3 and AIM2 inflammasomes, and reveal a similar requirement for ASC in caspase-1 autoprocessing by the NLRP1b inflammasome. 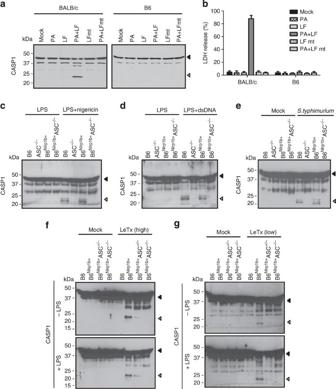Figure 1: ASC is critical for caspase-1 autoproteolysis by known inflammasomes. (a,b) BALB/c and B6 macrophages were treated with PA (10 μg) and/or wild-type LF (10 μg) and the enzymatically inactive LFE687Cmutant (LFmt) for 3 h, after which lysates were immunoblotted for caspase-1 (a) and culture supernatants analysed for LDH release (b). Data are shown as mean±s.d. from a single representative experiment of three experiments, with each condition performed in triplicate. (c–e) Lysates of B6, ASC−/−, B6Nlrp1b+and B6Nlrp1b+ASC−/−BMDMs were immunoblotted for caspase-1 after cells have been primed with 5 μg ml−1LPS for 3 h and subsequently stimulated with 20 μM nigericin for 60 min (c), pretreated with 5 μg ml−1LPS (3 h) and subsequently transfected with 1 μg dsDNA for 24 h (d) or infected withS. typhimurium(m.o.i. 10) for 3 h (e). (f,g) B6, B6Nlrp1b+, B6Nlrp1b+ASC+/−and B6Nlrp1b+ASC−/−BMDMs were left untreated or pretreated with 5 μg ml−1LPS for 3 h prior to being exposed to different concentrations of LeTx (f, 10 μg PA+10 μg LF) or (g, 500 ng PA+250 ng LF) for another 3 h. Cell lysates were immunoblotted for caspase-1. Data are representative of results from three experiments. Figure 1: ASC is critical for caspase-1 autoproteolysis by known inflammasomes. ( a , b ) BALB/c and B6 macrophages were treated with PA (10 μg) and/or wild-type LF (10 μg) and the enzymatically inactive LF E687C mutant (LFmt) for 3 h, after which lysates were immunoblotted for caspase-1 ( a ) and culture supernatants analysed for LDH release ( b ). Data are shown as mean±s.d. from a single representative experiment of three experiments, with each condition performed in triplicate. ( c – e ) Lysates of B6, ASC −/− , B6 Nlrp1b+ and B6 Nlrp1b+ ASC −/− BMDMs were immunoblotted for caspase-1 after cells have been primed with 5 μg ml −1 LPS for 3 h and subsequently stimulated with 20 μM nigericin for 60 min ( c ), pretreated with 5 μg ml −1 LPS (3 h) and subsequently transfected with 1 μg dsDNA for 24 h ( d ) or infected with S. typhimurium (m.o.i. 10) for 3 h ( e ). ( f , g ) B6, B6 Nlrp1b+ , B6 Nlrp1b+ ASC +/− and B6 Nlrp1b+ ASC −/− BMDMs were left untreated or pretreated with 5 μg ml −1 LPS for 3 h prior to being exposed to different concentrations of LeTx ( f , 10 μg PA+10 μg LF) or ( g , 500 ng PA+250 ng LF) for another 3 h. Cell lysates were immunoblotted for caspase-1. Data are representative of results from three experiments. Full size image NLRP1b-driven pyroptosis is unaffected by ASC deletion To understand the role of ASC in cell death induction, LPS-primed B6, ASC −/− , B6 Nlrp1b+ and B6 Nlrp1b+ ASC −/− macrophages were stimulated with the NLRP3 inflammasome activator nigericin, or transfected with dsDNA to trigger the AIM2 inflammasome. Both nigericin and dsDNA transfection triggered cell death levels in B6 macrophages that were comparable to those of B6 Nlrp1b+ cells ( Fig. 2a,b ). Nigericin- and dsDNA-induced cell lysis was markedly—albeit not fully—inhibited in ASC −/− and B6 Nlrp1b+ ASC −/− macrophages, suggesting that ASC is partially required for pyroptosis induction by the NLRP3 and AIM2 inflammasomes, respectively. As expected [17] , [18] , S. typhimurium infection induced similar pyroptosis levels in B6 and ASC −/− macrophages, as well as in B6 Nlrp1b+ and B6 Nlrp1b+ ASC −/− cells ( Fig. 2c ), indicating that ASC is dispensable for NLRC4 inflammasome-mediated pyroptosis induction. ASC also is dispensable for pyroptosis induction by the NLRP1b inflammasome because cell death of macrophages exposed for 3 h to either high ( Fig. 2d ) or low ( Fig. 2e ) concentrations of LeTx was independent of ASC expression. Further titration of the LeTx concentration reduced cell death responses in ASC-expressing and ASC-deficient BMDMs to a similar extent, confirming that ASC is not required for LeTx-induced pyroptosis ( Supplementary Fig. 2a ). As expected, the caspase-1 inhibitor Ac-YVAD-cmk inhibited LeTx-induced caspase-1 autoproteolysis in B6 Nlrp1b+ cells ( Supplementary Fig. 2b ). Although caspase-1 was not processed in LeTx-treated B6 Nlrp1b+ ASC −/− macrophages ( Fig. 1f,g ), these cells were equally sensitive to cell death blockade by Ac-YVAD-cmk as B6 Nlrp1b+ cells expressing ASC ( Fig. 2f,g ), suggesting that caspase-1 is active and induces pyroptosis in LeTx-treated macrophages irrespective of its processing status. Indeed, Ac-YVAD-cmk-mediated protection against pyroptosis was due to caspase-1 inhibition because LeTx-induced pyroptosis was abrogated in B6 Nlrp1b+ Casp1 −/− macrophages ( Fig. 2h ). Notably, B6 macrophages (lacking a functional NLRP1b allele) that were exposed to LeTx for 3 h were resistant to pyroptosis induction ( Fig. 2d,e ), but extended incubation for 24 h triggered significant cell lysis with levels reaching about half of those seen in cells expressing a functional NLRP1b allele regardless of their ASC expression status ( Fig. 2i,j ). This suggests that macrophage cell death uniquely relies on the NLRP1b inflammasome during initial phases of LeTx intoxication, whereas sustained LeTx exposure triggers additional inflammasome-independent cell death mechanisms at later time points. Together, these results demonstrate that ASC is dispensable for early NLRP1b-mediated cell death induction in LeTx-intoxicated macrophages. 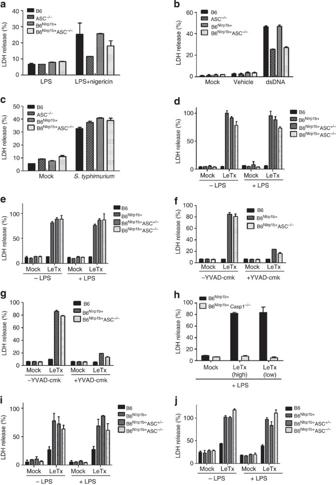Figure 2: Role of ASC in pyroptosis induction by distinct inflammasomes. (a–c) B6, ASC−/−, B6Nlrp1b+and B6Nlrp1b+ASC−/−BMDMs were primed with 5 μg ml−1LPS for 3 h and subsequently stimulated with 20 μM nigericin for 60 min (a) or transfected with 1 μg dsDNA for 24 h (b), or infected withS. typhimurium(m.o.i. 10) for 3 h in the absence of LPS priming (c) before LDH levels were determined in culture supernatants. (d,e) B6, B6Nlrp1b+, B6Nlrp1b+ASC+/−and B6Nlrp1b+ASC−/−BMDMs were left untreated or pretreated with 5 μg ml−1LPS for 3 h prior to being exposed to different concentrations of LeTx (d, 10 μg PA+10 μg LF) or (e, 500 ng PA+250 ng LF) for another 3 h before LDH levels were determined in culture supernatants. (f,g) LPS-primed B6, B6Nlrp1b+and B6Nlrp1b+ASC−/−BMDMs were pre-incubated with 50 μM ac-YVAD-cmk for 30 min prior to LeTx treatment for 3 h (f, 10 μg PA+10 μg LF;g, 500 ng PA+250 ng LF) before LDH levels were determined in culture supernatants. (h) B6Nlrp1b+and B6Nlrp1b+Casp1−/−BMDMs were primed with 5 μg ml−1LPS for 3 h before LeTx treatment (high, 10 μg PA+10 μg LF; low, 500 ng PA+250 ng LF) for another 3 h followed by LDH measurement in culture supernatants. (i,j) B6, B6Nlrp1b+, B6Nlrp1b+ASC+/−and B6Nlrp1b+ASC−/−BMDMs were left untreated or primed with 5 μg ml−1LPS for 3 h before LeTx treatment (i, 10 μg PA+10 μg LF;j, 500 ng PA+250 ng LF) for 24 h before LDH levels were determined in culture supernatants. Data are shown as mean±s.d. from a single representative experiment of three experiments, with each condition performed in triplicate. Figure 2: Role of ASC in pyroptosis induction by distinct inflammasomes. ( a – c ) B6, ASC −/− , B6 Nlrp1b+ and B6 Nlrp1b+ ASC −/− BMDMs were primed with 5 μg ml −1 LPS for 3 h and subsequently stimulated with 20 μM nigericin for 60 min ( a ) or transfected with 1 μg dsDNA for 24 h ( b ), or infected with S. typhimurium (m.o.i. 10) for 3 h in the absence of LPS priming ( c ) before LDH levels were determined in culture supernatants. ( d , e ) B6, B6 Nlrp1b+ , B6 Nlrp1b+ ASC +/− and B6 Nlrp1b+ ASC −/− BMDMs were left untreated or pretreated with 5 μg ml −1 LPS for 3 h prior to being exposed to different concentrations of LeTx ( d , 10 μg PA+10 μg LF) or ( e , 500 ng PA+250 ng LF) for another 3 h before LDH levels were determined in culture supernatants. ( f , g ) LPS-primed B6, B6 Nlrp1b+ and B6 Nlrp1b+ ASC −/− BMDMs were pre-incubated with 50 μM ac-YVAD-cmk for 30 min prior to LeTx treatment for 3 h ( f , 10 μg PA+10 μg LF; g , 500 ng PA+250 ng LF) before LDH levels were determined in culture supernatants. ( h ) B6 Nlrp1b+ and B6 Nlrp1b+ Casp1 −/− BMDMs were primed with 5 μg ml −1 LPS for 3 h before LeTx treatment (high, 10 μg PA+10 μg LF; low, 500 ng PA+250 ng LF) for another 3 h followed by LDH measurement in culture supernatants. ( i , j ) B6, B6 Nlrp1b+ , B6 Nlrp1b+ ASC +/− and B6 Nlrp1b+ ASC −/− BMDMs were left untreated or primed with 5 μg ml −1 LPS for 3 h before LeTx treatment ( i , 10 μg PA+10 μg LF; j , 500 ng PA+250 ng LF) for 24 h before LDH levels were determined in culture supernatants. Data are shown as mean±s.d. from a single representative experiment of three experiments, with each condition performed in triplicate. Full size image ASC is dispensable for lethal toxin-induced IL-1β secretion Our results showed that LeTx-induced pyroptosis was normal in ASC-deficient macrophages although caspase-1 autoproteolysis was abolished, implying that caspase-1 zymogen recruitment in the NLRP1b inflammasome is sufficient for gaining enzymatic activity in the absence of caspase-1 autoproteolysis. Apart from pyroptotic cell death, inflammasomes mediate secretion of mature IL-1β [20] . We therefore examined the role of ASC in IL-1β secretion by distinct inflammasomes. The NLRP3 inflammasome stimulus nigericin induced significant IL-1β secretion from LPS-primed B6 and B6 Nlrp1b+ macrophages, and these responses were abrogated in ASC −/− and B6 Nlrp1b+ ASC −/− macrophages ( Fig. 3a ). Similarly, dsDNA-mediated activation of the AIM2 inflammasome induced potent secretion of IL-1β in ASC-expressing macrophages, but not in cells lacking ASC ( Fig. 3b ). Also, NLRC4 inflammasome-mediated cytokine secretion by S. typhimurium -infected macrophages required ASC ( Fig. 3c ). In sharp contrast, heterozygous and homozygous deletion of ASC failed to affect IL-1β secretion by LPS-primed B6 Nlrp1b+ macrophages that have been treated with a high concentration of LeTx ( Fig. 3d,e ). As expected, B6 macrophages failed to secrete mature IL-1β into the culture medium, in agreement with the requirement for a functional NLRP1b allele. ASC deletion partially affected cytokine secretion from cells exposed to a lower concentration of LeTx for 3 h, although B6 Nlrp1b+ ASC +/− and B6 Nlrp1b+ ASC −/− macrophages still secreted significant amounts of IL-1β ( Fig. 3f,g ). Similar results were obtained when macrophages were treated for 24 h: ASC-deficient cells secreted normal IL-1β levels when exposed to a high dose of LeTx, and reduced levels with a low LeTx concentration ( Supplementary Fig. 3a,b ). The inflammatory caspase inhibitor Ac-YVAD-cmk efficiently blocked LeTx-induced cytokine secretion ( Fig. 3h,i ), confirming that LeTx-induced IL-1β secretion required caspase-1. In agreement, genetic deletion of caspase-1 abrogated LeTx-induced IL-1β secretion from LPS-primed B6 Nlrp1b+ Casp1 −/− macrophages ( Fig. 3j,k ). A recent report showed that enteropathogen-induced caspase-1 autoproteolysis and IL-1β secretion by the non-canonical Nlrp3 inflammasome required caspase-11, and that 129S macrophages are naturally deficient in caspase-11 expression [21] . However, LeTx induced caspase-1 autoproteolysis ( Fig. 3l ), IL-1β ( Fig. 3m ) and IL-18 ( Fig. 3n ) secretion in LPS-primed 129S macrophages, indicating that caspase-11 is dispensable for LeTx-induced activation of the NLRP1b inflammasome. Together, these results indicate that, unlike its role in the NLRP3, AIM2 and NLRC4 inflammasomes, ASC is not critical for cytokine secretion by the NLRP1b inflammasome, although it enhances cytokine secretion at lower LeTx concentrations. 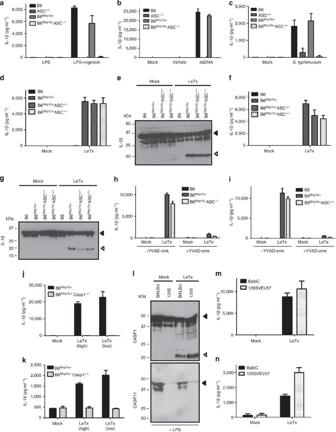Figure 3: ASC is dispensable for IL-1β secretion by the NLRP1b inflammasome. (a–c) B6, ASC−/−, B6Nlrp1b+and B6Nlrp1b+ASC−/−BMDMs were primed with 5 μg ml−1LPS for 3 h and subsequently stimulated with 20 μM nigericin for 60 min (a) or transfected with 1 μg dsDNA for 24 h (b) or infected withS. typhimurium(m.o.i. 10) for 3 h in the absence of LPS priming (c) before secreted IL-1β levels were determined in culture supernatants. (d–g) B6, B6Nlrp1b+, B6Nlrp1b+ASC+/−and B6Nlrp1b+ASC−/−BMDMs were left untreated or pretreated with 5 μg ml−1LPS for 3 h prior to being exposed to different concentrations of LeTx (d,e, 10 μg PA+10 μg LF) or (f,g, 500 ng PA+250 ng LF) for another 3 h. Secreted IL-1β levels were determined in culture supernatants by ELISA and lysates were immunoblotted for IL-1β. (h,i) LPS-primed B6, B6Nlrp1b+and B6Nlrp1b+ASC−/−BMDMs were pre-incubated with 50 μM ac-YVAD-cmk for 30 min prior to LeTx treatment for 3 h (h, 10 μg PA+10 μg LF;i, 500 ng PA+250 ng LF). Secreted IL-1β levels were determined in culture supernatants. (j,k) B6Nlrp1b+and B6Nlrp1b+Casp1−/−BMDMs were primed with 5 μg ml−1LPS for 3 h followed by LeTx treatment (high, 10 μg PA+10 μg LF; low, 500 ng PA+250 ng LF) for another 3 h. Levels of secreted IL-1β (j) and IL-18 (k) were determined in culture supernatants. (l–n) BALB/C and 129SVEV57 BMDMs were primed with 5 μg ml−1LPS for 3 h prior to LeTx treatment (10 μg PA+10 μg LF) for another 3 h. Lysates were immunoblotted for the indicated proteins (l) and secreted IL-1β and IL-18 were determined in culture supernatants by ELISA (m,n). Data are shown as mean±s.d. from a single representative experiment of three experiments, with each condition performed in triplicate. Figure 3: ASC is dispensable for IL-1β secretion by the NLRP1b inflammasome. ( a – c ) B6, ASC −/− , B6 Nlrp1b+ and B6 Nlrp1b+ ASC −/− BMDMs were primed with 5 μg ml −1 LPS for 3 h and subsequently stimulated with 20 μM nigericin for 60 min ( a ) or transfected with 1 μg dsDNA for 24 h ( b ) or infected with S. typhimurium (m.o.i. 10) for 3 h in the absence of LPS priming ( c ) before secreted IL-1β levels were determined in culture supernatants. ( d – g ) B6, B6 Nlrp1b+ , B6 Nlrp1b+ ASC +/− and B6 Nlrp1b+ ASC −/− BMDMs were left untreated or pretreated with 5 μg ml −1 LPS for 3 h prior to being exposed to different concentrations of LeTx ( d , e , 10 μg PA+10 μg LF) or ( f , g , 500 ng PA+250 ng LF) for another 3 h. Secreted IL-1β levels were determined in culture supernatants by ELISA and lysates were immunoblotted for IL-1β. ( h , i ) LPS-primed B6, B6 Nlrp1b+ and B6 Nlrp1b+ ASC −/− BMDMs were pre-incubated with 50 μM ac-YVAD-cmk for 30 min prior to LeTx treatment for 3 h ( h , 10 μg PA+10 μg LF; i , 500 ng PA+250 ng LF). Secreted IL-1β levels were determined in culture supernatants. ( j , k ) B6 Nlrp1b+ and B6 Nlrp1b+ Casp1 −/− BMDMs were primed with 5 μg ml −1 LPS for 3 h followed by LeTx treatment (high, 10 μg PA+10 μg LF; low, 500 ng PA+250 ng LF) for another 3 h. Levels of secreted IL-1β ( j ) and IL-18 ( k ) were determined in culture supernatants. ( l – n ) BALB/C and 129SVEV57 BMDMs were primed with 5 μg ml −1 LPS for 3 h prior to LeTx treatment (10 μg PA+10 μg LF) for another 3 h. Lysates were immunoblotted for the indicated proteins ( l ) and secreted IL-1β and IL-18 were determined in culture supernatants by ELISA ( m , n ). Data are shown as mean±s.d. from a single representative experiment of three experiments, with each condition performed in triplicate. Full size image ASC and functional NLRP1b are essential for speck formation ASC mediates the assembly of a single macromolecular perinuclear structure referred to as ‘speck’ in macrophages treated with stimuli of the NLRP3 (ref. 22 ), NLRC4 (ref. 17 ) and AIM2 inflammasomes [23] . These specks have been associated with efficient cytokine secretion by the NLRC4 inflammasome [17] , and cell death induction by the NLRP3 inflammasome [22] . However, it is not known whether specks are formed under conditions of NLRP1b inflammasome activation. To examine LeTx-induced speck formation and its requirements, we analysed the subcellular localization of ASC and caspase-1 in B6, B6 Nlrp1b+ and B6 Nlrp1b+ ASC −/− macrophages by immunostaining before and after LeTx treatment. As expected, ASC mainly localized to the nuclear compartment of naive wild-type cells, and the immunofluorescent signal was largely lost in ASC cells ( Supplementary Fig. 4a ). Similarly, the caspase-1-specific antibody failed to stain caspase-1-deficient macrophages ( Supplementary Fig. 4b ), demonstrating specificity of the respective antibodies. LeTx treatment induced formation of a single, brightly stained perinuclear speck that contained both ASC and caspase-1 in some B6 Nlrp1b+ macrophages ( Fig. 4a,b ). Notably, these specks failed to form in LeTx-treated B6 and B6 Nlrp1b+ ASC −/− macrophages ( Fig. 4a,b ), demonstrating that a functional NLRP1b allele and ASC expression are essential for LeTx-induced speck formation. 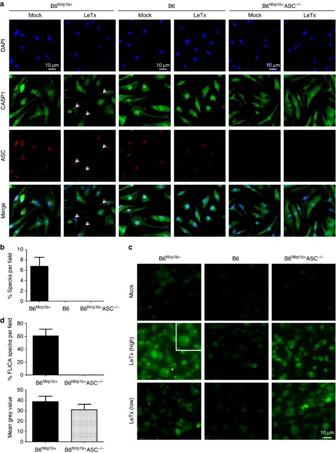Figure 4: ASC is critical for LeTx-induced speck formation. (a) B6, B6Nlrp1b+and B6Nlrp1b+ASC−/−BMDMs were grown on coverslips and treated with LeTx (10 μg PA and LF, respectively) for 60 min after which cells were fixed in 4% paraformaldehyde and immunostained for ASC (red) and caspase-1 (green). DAPI (blue) was included to localize nuclei. Arrows indicate specks. Confocal micrographs were acquired at × 60 magnification. (b) Quantification of specks per field. (c) B6, B6Nlrp1b+and B6Nlrp1b+ASC−/−BMDMs that were stimulated with LeTx (high, 10 μg PA+10 μg LF; low, 500 ng PA+250 ng LF) for 30 min, and then incubated with the active caspase-1 Fam-YVAD-fmk FLICA probe for 45 min before fluorescent micrographs were acquired at × 20 magnification. * indicates magnified area. (d) Quantification of FLICA-positive cells/field and mean grey value. Data are representative of results from two independent experiments and quantification data are presented as mean±s.d. from a single representative experiment. Figure 4: ASC is critical for LeTx-induced speck formation. ( a ) B6, B6 Nlrp1b+ and B6 Nlrp1b+ ASC −/− BMDMs were grown on coverslips and treated with LeTx (10 μg PA and LF, respectively) for 60 min after which cells were fixed in 4% paraformaldehyde and immunostained for ASC (red) and caspase-1 (green). DAPI (blue) was included to localize nuclei. Arrows indicate specks. Confocal micrographs were acquired at × 60 magnification. ( b ) Quantification of specks per field. ( c ) B6, B6 Nlrp1b+ and B6 Nlrp1b+ ASC −/− BMDMs that were stimulated with LeTx (high, 10 μg PA+10 μg LF; low, 500 ng PA+250 ng LF) for 30 min, and then incubated with the active caspase-1 Fam-YVAD-fmk FLICA probe for 45 min before fluorescent micrographs were acquired at × 20 magnification. * indicates magnified area. ( d ) Quantification of FLICA-positive cells/field and mean grey value. Data are representative of results from two independent experiments and quantification data are presented as mean±s.d. from a single representative experiment. Full size image To analyse whether these ASC specks contained active caspase-1, mock- and LeTx-treated macrophages were analysed by fluorescence microscopy using the active caspase-1 FLICA probe. The emission filter used to detect the FLICA signal passed a weak cellular autofluorescence background in mock-treated macrophages that was not due to the active caspase-1 probe because a similar background staining was evident in cells not exposed to the FLICA reagent ( Supplementary Fig. 4c ). In agreement with NLRP1b inflammasome-dependent caspase-1 activation, the FLICA signal increased significantly in B6 Nlrp1b+ macrophages upon treatment with a high or low concentration of LeTx, but not in B6 macrophages lacking a functional NLRP1b allele ( Fig. 4c ). Notably, LeTx-treated B6 Nlrp1b+ macrophages contained active caspase-1 in a single bright perinuclear speck and diffusely throughout the cell ( Fig. 4c,d ). Whereas diffuse active caspase-1 staining was retained in LeTx-treated B6 Nlrp1b+ ASC −/− macrophages, its focal localization in perinuclear specks was abrogated ( Fig. 4c,d ). Together, these results show that a functional NLRP1b allele and ASC expression are required for speck assembly and recruitment of active caspase-1 to these specks in LeTx-intoxicated macrophages. Role of ASC in lethal toxin-challenged BALB/c macrophages Our results showed that ASC is required for caspase-1 autoprocessing and speck formation in LeTx-treated B6 Nlrp1b+ macrophages, but not for pyroptosis induction and IL-1β secretion. Although we assured that NLRP1b transcript levels in these cells were similar to those of endogenous NLRP1b in 129S macrophages ( Supplementary Fig. 1b ), we wanted to confirm our findings in the absence of transgenic NLRP1b expression. To this end, ASC −/− mice were bred to a BALB/c genetic background for 10 generations before BMDMs from the resulting ASC −/− mice were intoxicated with LeTx. In agreement with our observations in B6 Nlrp1b+ ASC −/− macrophages, lysates of BALB/c macrophages showed potent caspase-1 autoprocessing in response to LeTx treatment, and this was abrogated in the absence of ASC ( Fig. 5a ). As expected, specks were formed in LeTx-treated wildtype BALB/c macrophages, but not in cells lacking ASC ( Supplementary Fig. 5 ). Despite defective caspase-1 autoproteolysis, pyroptosis induction in BALB/c ASC −/− macrophages treated with high or low concentrations of LeTx was similar to that of ASC-expressing BALB/c cells, respectively ( Fig. 5b,c ). Moreover, as we showed earlier for B6 Nlrp1b+ ASC −/− cells ( Fig. 3d ), secretion of IL-1β in response to high concentration of LeTx was similar in ASC-expressing and ASC-deficient BALB/c macrophages ( Fig. 5d,e ), while cytokine secretion was partially affected in ASC −/− cells when intoxicated with a lower concentration of LeTx ( Fig. 5d,f ). As in B6 Nlrp1b+ Casp1 −/− macrophages, deletion of caspase-1 in BALB/c mice prevented LeTx-induced macrophage pyroptosis ( Fig. 5g ), and secretion of IL-1β and IL-18 ( Fig. 5h,i ). Together, these results confirm that LeTx induces pyroptosis and cytokine production in the absence of ASC-mediated caspase-1 autoprocessing, and that ASC specifically enhances cytokine production at lower LeTx concentrations. 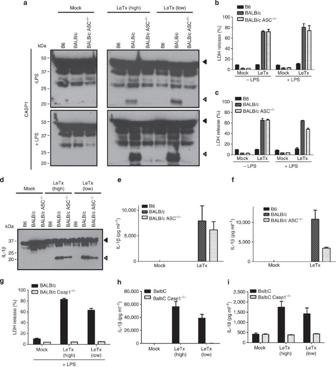Figure 5: ASC-deficiency in BALB/c macrophages prevents LeTx-induced caspase-1 autoproteolysis but not pyroptosis and IL-1β secretion. (a–f) B6, BALB/c and BALB/c ASC−/−BMDMs were left untreated or pretreated with 5 μg ml−1LPS for 3 h before incubation with LeTx (high, 10 μg PA+10 μg LF; low, 500 ng PA+250 ng LF) for another 3 h. Cell lysates were immunoblotted for caspase-1 and IL-1β (a,d) and culture supernatants were analysed for LDH (b,c) and secreted IL-1β (e,f). (g–i) BALB/c and BALB/c Casp1−/−BMDMs were primed with 5 μg ml−1LPS for 3 h followed by LeTx treatment (high, 10 μg PA+10 μg LF; low, 500 ng PA+250 ng LF) for another 3 h. Levels of LDH (g) and secreted IL-1β (h) and IL-18 (i) were determined in culture supernatants. Data are representative of results from three experiments, and cytokine and LDH data are presented as mean±s.d. from a single representative experiment, with each condition performed in triplicate. Figure 5: ASC-deficiency in BALB/c macrophages prevents LeTx-induced caspase-1 autoproteolysis but not pyroptosis and IL-1β secretion. ( a – f ) B6, BALB/c and BALB/c ASC −/− BMDMs were left untreated or pretreated with 5 μg ml −1 LPS for 3 h before incubation with LeTx (high, 10 μg PA+10 μg LF; low, 500 ng PA+250 ng LF) for another 3 h. Cell lysates were immunoblotted for caspase-1 and IL-1β ( a , d ) and culture supernatants were analysed for LDH ( b , c ) and secreted IL-1β ( e , f ). ( g – i ) BALB/c and BALB/c Casp1 −/− BMDMs were primed with 5 μg ml −1 LPS for 3 h followed by LeTx treatment (high, 10 μg PA+10 μg LF; low, 500 ng PA+250 ng LF) for another 3 h. Levels of LDH ( g ) and secreted IL-1β ( h ) and IL-18 ( i ) were determined in culture supernatants. Data are representative of results from three experiments, and cytokine and LDH data are presented as mean±s.d. from a single representative experiment, with each condition performed in triplicate. Full size image Active caspase-1 is ubiquitinated independently of ASC Our results suggest that NLRP1b and caspase-1 assemble a functional inflammasome independently of ASC. In agreement, caspase-1 was shown to specifically co-precipitate NLRP1b when ectopically expressed, suggesting that caspase-1 and NLRP1b interact directly and that ASC is dispensable for this interaction [13] . Interestingly, caspase-1 activation in B6 Nlrp1b+ macrophages that were treated with either a high ( Fig. 6a ) or low ( Fig. 6b ) concentration of LeTx was consistently associated with the appearance of high-molecular weight species that are indicative of caspase-1 post-translational modification. LeTx-induced caspase-1 modification required a functional NLRP1b allele, but was independent of LPS priming, ASC expression and caspase-1 autoproteolysis ( Fig. 6a,b ). The high-molecular weight bands represented modified caspase-1 species because LeTx-induced caspase-1 immunoreactive bands were apparent in lysates of intoxicated B6 Nlrp1b+ and BALB/c macrophages, but not in the corresponding LeTx-treated caspase-1-deficient cells ( Fig. 6c,d ). Stimulus-induced caspase-1 modification was not limited to the NLRP1b inflammasome because modified caspase-1 also was observed in LPS-primed macrophages that were treated with the NLRP3 stimuli ATP and nigericin ( Fig. 6e ), in B6 macrophages that were infected with Francisella tularensis to activate the AIM2 inflammasome ( Fig. 6f ), and in macrophages infected with different MOIs of the NLRC4 inflammasome-activating pathogen S. typhimurium ( Fig. 6g ). Inflammasome-induced caspase-1 modification required caspase-1 enzymatic activity because Ac-YVAD-cmk inhibited LeTx-induced caspase-1 modification in both B6 Nlrp1b+ ( Fig. 6h ) and B6 Nlrp1b+ ASC −/− ( Fig. 6i ) macrophages. We next immunoprecipitated caspase-1 from LeTx-challenged and LPS+ATP-treated macrophages to characterize the molecular identity of the caspase-1 post-translational modification. These studies revealed caspase-1 to be ubiquitinated under conditions promoting its activation by the NLRP1b and NLRP3 inflammasomes, respectively ( Fig. 6j,k and Supplementary Fig. 6 ). In addition, we showed that LeTx-induced caspase-1 ubiquitination required NLRP1b and caspase-1 enzymatic activity, while ASC and caspase-1 autoproteolysis were dispensable. 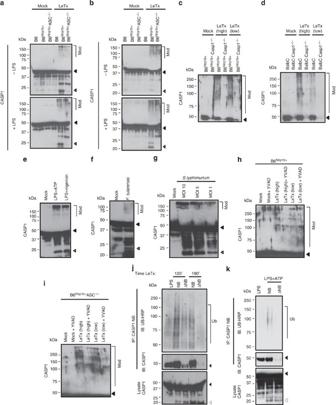Figure 6: ASC is dispensable for post-translational modification of active caspase-1. (a,b) B6, B6Nlrp1b+and B6Nlrp1b+ASC−/−BMDMs were left untreated or pretreated with 5 μg ml−1LPS for 3 h prior to being exposed to different concentrations of LeTx (a, 10 μg PA+10 μg LF) or (b, 500 ng PA+250 ng LF) for another 3 h. Cell lysates were immunoblotted for caspase-1. (c,d) B6Nlrp1b+and B6Nlrp1b+Casp1−/−(c), or BALB/c and BALB/c Casp1−/−BMDMs (d) were treated with 5 μg ml−1LPS for 3 h and subsequently exposed to 10 μg PA+10 μg LF (high) or 500 ng PA+250 ng LF (low) for another 3 h. Cell lysates were immunoblotted for caspase-1. (e–g) Lysates of B6 BMDMs were immunoblotted for caspase-1 after cells have been primed with 5 μg ml−1LPS for 3 h and subsequently stimulated with 5 mM ATP or 20 μM nigericin for 30 min (e), infected withF. tularensis(m.o.i. 30) for 3 h (f), or infected withS. typhimurium(m.o.i. 10, 5 and 1) for 3 h (g). (h,i) LPS-primed B6Nlrp1b+(h) and B6Nlrp1b+ASC−/−(i) BMDMs were pretreated with 50 μM Ac-YVAD-cmk for 30 min prior to being exposed to 10 μg PA+10 μg LF (High), or 500 ng PA+250 ng LF (Low) for another 3 h. Cell lysates were immunoblotted for caspase-1. (j,k) LPS-primed BALB/c BMDMs were exposed to 500 ng PA+250 ng LF ml−1for 120 or 190 min, respectively (j), or treated with 5 mM ATP for 30 min (k) before caspase-1 was immunoprecipitated using caspase-1 nanobody clone R2S40. Immunoprecipitates and lysates were immunoblotted for the indicated proteins. Data are representative of results from at least three independent experiments. Figure 6: ASC is dispensable for post-translational modification of active caspase-1. ( a , b ) B6, B6 Nlrp1b+ and B6 Nlrp1b+ ASC −/− BMDMs were left untreated or pretreated with 5 μg ml −1 LPS for 3 h prior to being exposed to different concentrations of LeTx ( a , 10 μg PA+10 μg LF) or ( b , 500 ng PA+250 ng LF) for another 3 h. Cell lysates were immunoblotted for caspase-1. ( c , d ) B6 Nlrp1b+ and B6 Nlrp1b+ Casp1 −/− ( c ), or BALB/c and BALB/c Casp1 −/− BMDMs ( d ) were treated with 5 μg ml −1 LPS for 3 h and subsequently exposed to 10 μg PA+10 μg LF (high) or 500 ng PA+250 ng LF (low) for another 3 h. Cell lysates were immunoblotted for caspase-1. ( e – g ) Lysates of B6 BMDMs were immunoblotted for caspase-1 after cells have been primed with 5 μg ml −1 LPS for 3 h and subsequently stimulated with 5 mM ATP or 20 μM nigericin for 30 min ( e ), infected with F. tularensis (m.o.i. 30) for 3 h ( f ), or infected with S. typhimurium (m.o.i. 10, 5 and 1) for 3 h ( g ). ( h , i ) LPS-primed B6 Nlrp1b+ ( h ) and B6 Nlrp1b+ ASC −/− ( i ) BMDMs were pretreated with 50 μM Ac-YVAD-cmk for 30 min prior to being exposed to 10 μg PA+10 μg LF (High), or 500 ng PA+250 ng LF (Low) for another 3 h. Cell lysates were immunoblotted for caspase-1. ( j , k ) LPS-primed BALB/c BMDMs were exposed to 500 ng PA+250 ng LF ml −1 for 120 or 190 min, respectively ( j ), or treated with 5 mM ATP for 30 min ( k ) before caspase-1 was immunoprecipitated using caspase-1 nanobody clone R2S40. Immunoprecipitates and lysates were immunoblotted for the indicated proteins. Data are representative of results from at least three independent experiments. Full size image In vivo role of ASC in the NLRP1b inflammasome LeTx injection in vivo induces many symptoms associated with anthrax spore infection, including inflammation and death [9] . To address the physiological relevance of NLRP1b inflammasome signalling in the absence of ASC-dependent caspase-1 autoproteolysis, groups of B6, B6 Nlrp1b+ and B6 Nlrp1b+ ASC −/− mice were injected intraperitoneally with LeTx (100 μg g −1 PA and LF, respectively). Western blot analysis of whole spleen lysates prepared 3 h post injection showed that LeTx efficiently induced caspase-1 autoprocessing in B6 Nlrp1b+ mice, but not in B6 mice ( Fig. 7a ). As in macrophages, these results demonstrate that a functional NLRP1b allele is critical for caspase-1 autoprocessing in LeTx-induced animals. Caspase-1 cleavage also was abrogated in B6 Nlrp1b+ mice deficient in ASC expression ( Fig. 7a ), confirming the critical role of ASC in LeTx-induced caspase-1 autoproteolysis in vivo . To study the in vivo role of NLRP1b and ASC in LeTx-induced cell death, serum was analysed for release of HMGB1, a danger signal released by dying cells during trauma and infection [20] . Concurrent with our observation that LeTx-induced macrophage cell death in a NLRP1b-dependent and ASC-independent manner, LeTx-induced levels of circulating HMGB1 were similarly elevated in B6 Nlrp1b+ and B6 Nlrp1b+ ASC −/− mice, whereas levels of circulating HMGB1 in serum samples of unchallenged B6 Nlrp1b+ and B6 Nlrp1b+ ASC −/− mice and LeTx-challenged B6 mice were below the detection limit of the antibody ( Fig. 7b ). LeTx-induced secretion of IL-1β ( Fig. 7c ) and IL-18 ( Fig. 7d ) also required a functional NLRP1b allele because B6 mice failed to release these inflammasome-dependent cytokines when challenged with LeTx. Notably, B6 Nlrp1b+ ASC −/− mice contained high levels of circulating IL-1β and IL-18, although these were statistically lower than those of B6 Nlrp1b+ littermates ( Fig. 7c,d ). These results confirm that ASC is not essential but contributes to NLRP1b-mediated cytokine secretion in vivo . To address the importance of NLRP1b- and ASC-mediated signalling for LeTx-induced lethality, cohorts of mice were challenged with a lethal dose of LeTx (200 μg g −1 PA and LF, respectively). In agreement with published reports suggesting that LeTx susceptibility of inbred mouse and rat strains correlated with the rodent chromosomal loci encoding NLRP1b [24] , [25] , LeTx-challenged B6 mice resisted significantly longer to LeTx-induced death than B6 mice expressing a functional NLRP1b allele ( Fig. 7e ). Similarly, B6 Nlrp1b+ ASC −/− mice succumbed much faster to LeTx challenge than B6 mice, although they died with similar kinetics as B6 Nlrp1b+ littermates ( Fig. 7e ). Together, these findings suggest a mechanistic model in which functional NLRP1b directly (independently of ASC) recruits procaspase-1 zymogens to assemble octa- or heptameric NLRP1b inflammasomes upon detection of LF metalloprotease activity in the cytosol ( Fig. 7f ). Procaspase-1 is likely recruited to these complexes by means of direct homotypic interactions between its prodomain and the C-terminal CARD of NLRP1b. Inflammasome complex assembly may induce conformational changes in procaspase-1 that allow it to gain enzymatic activity and cleave IL-1β, IL-18 and yet unknown substrates leading to cell death. ASC-mediated oligomerization of multiple (ASC-free) NLRP1b inflammasomes induces formation of a single, large perinuclear speck in which procaspase-1 undergoes autoproteolysis, which may serve to stabilize the active protease and further enhance cytokine production ( Fig. 7f ). 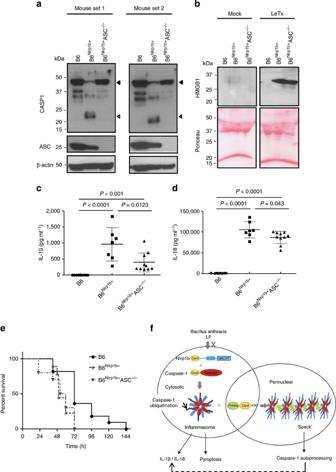Figure 7:In vivorole of ASC in LeTx-challenged mice. (a–d) B6 (n=9), B6Nlrp1b+(n=7) and B6Nlrp1b+ASC−/−mice (n=10) were injected intraperitoneally with LeTx (100 μg PA and LF, respectively), and spleen and serum were collected 3 h later. Spleen (a) and serum samples (b) were immunoblotted for the indicated proteins. Ponceau staining was performed as loading control for serum samples (b). Circulating IL-1β (c) and IL-18 (d) levels in serum was determined by ELISA, with each dot representing an individual mouse. Statistical significance was determined by Student’st-test andP-values are indicated. (e) B6 (n=11), B6Nlrp1b+(n=9) and B6Nlrp1b+ASC−/−(n=10) mice were injected intraperitoneally with a lethal dose of LeTx (200 μg PA and LF, respectively) and survival was monitored over time. Statistical significance was determined by Kaplan–Meier analysis andP-values were as follows: B6 vs B6Nlrp1b+,P=0.0096; B6 vs B6Nlrp1b+ASC−/−,P=0.0086; B6Nlrp1b+vs B6Nlrp1b+ASC−/−,P=0.79 (non-significant). (f) Schematic model depicting the putative role of ASC in Nlrp1b inflammasome signalling in LeTx-challenged macrophages and mice. Figure 7: In vivo role of ASC in LeTx-challenged mice. ( a – d ) B6 ( n =9), B6 Nlrp1b+ ( n =7) and B6 Nlrp1b+ ASC −/− mice ( n =10) were injected intraperitoneally with LeTx (100 μg PA and LF, respectively), and spleen and serum were collected 3 h later. Spleen ( a ) and serum samples ( b ) were immunoblotted for the indicated proteins. Ponceau staining was performed as loading control for serum samples ( b ). Circulating IL-1β ( c ) and IL-18 ( d ) levels in serum was determined by ELISA, with each dot representing an individual mouse. Statistical significance was determined by Student’s t -test and P -values are indicated. ( e ) B6 ( n =11), B6 Nlrp1b+ ( n =9) and B6 Nlrp1b+ ASC −/− ( n =10) mice were injected intraperitoneally with a lethal dose of LeTx (200 μg PA and LF, respectively) and survival was monitored over time. Statistical significance was determined by Kaplan–Meier analysis and P -values were as follows: B6 vs B6 Nlrp1b+ , P =0.0096; B6 vs B6 Nlrp1b+ ASC −/− , P =0.0086; B6 Nlrp1b+ vs B6 Nlrp1b+ ASC −/− , P =0.79 (non-significant). ( f ) Schematic model depicting the putative role of ASC in Nlrp1b inflammasome signalling in LeTx-challenged macrophages and mice. Full size image LeTx is lethal to nearly all mammalian species, and is considered the major virulence factor of B. anthracis because in vivo LeTx intoxication mimics disease progression in mammalian hosts that have been infected with B. anthracis spores, the causative agent of anthrax [9] , [26] . Depending on the route of infection, resident macrophages of respectively the lung, intestine or skin are targeted by B. anthracis spores for germination and bacterial replication, which may result in systemic dispersion of the infectious agent into the bloodstream [27] , [28] . Macrophages from inbred mouse strain respond differentially to LeTx intoxication. Those that express a functional NLRP1b allele (such as 129S and BALB/c) induce rapid cell lysis, whereas those of resistant mouse strains (such as C57BL/6) encode mutated NLRP1b alleles [8] . Moreover, NLRP1b-induced macrophage cell death is—at least partially—correlated with the relative susceptibility of inbred mouse and rat strains to rapid LeTx-induced mortality in vivo [24] , [25] , [28] . Upon PA-mediated access to the cytosolic compartment of intoxicated macrophages, the LF zinc protease subunit of LeTx cleaves MKK proteins and currently unknown substrates [29] , [30] . The host’s immune system responds to LeTx proteolytic activity in the cytosol with assembly of the NLRP1b inflammasome, a protein complex that facilitates activation of the inflammatory cysteine protease caspase-1 (ref. 1 ). NLRP1b-activated caspase-1 converts the inflammatory cytokines IL-1β and IL-18 into their secreted bioactive forms, and induces pyroptotic cell death in sensitive macrophages [20] . However, the molecular composition and mechanisms by which the NLRP1b inflammasome controls caspase-1 activation, cytokine secretion and pyroptosis are unclear. Some reports relying on ectopic expression of inflammasome components suggested ASC to be dispensable for NLRP1b inflammasome signalling [12] , [13] , while other reports implicated ASC in NLRP1b inflammasome signalling [14] . Our analysis of LeTx-sensitive ASC-sufficient and -deficient cells and mice revealed that ASC was critical for particular, but not all, aspects of NLRP1b inflammasome signalling. Notably, co-incubation of recombinant human procaspase-1 and NLRP1 in vitro in the absence of ASC elicited caspase-1 autoproteolysis [31] , whereas our studies in ASC-deficient macrophages indicated ASC to be required for caspase-1 autoprocessing by the NLRP1b inflammasome. Moreover, using fluorescence and confocal microscopic analysis, we demonstrated that speck formation occurs in LeTx-treated macrophages, and that their assembly was strictly dependent on the expression of ASC and a functional NLRP1b allele. In addition, we showed that these specks correlated with focal localization of active caspase-1 in the perinuclear region of intoxicated wild-type cells. However, despite absent speck formation, ASC-deficient macrophages secreted significant amounts of IL-1β. In addition, ASC-deficient macrophages underwent normal LeTx-induced cell lysis. In contrast, both IL-1β secretion and pyroptosis were ablated in cells lacking a functional NLRP1b allele, or when caspase-1 activity was pharmacologically inhibited, confirming that these responses were dependent on a functional NLRP1b inflammasome. Given that ASC was critical for cytokine production by the latter complexes, these observations suggest that the NLRP1b inflammasome differs fundamentally from other known (NLRP3, NLRC4 and AIM2) inflammasomes. They also suggest that the functional NLRP1b inflammasome is a structure distinct from ASC specks because NLRP1b- and caspase-1-dependent cytokine secretion and pyroptosis occurred in the absence of the latter. Notably, despite significant induction of cell death and cytokine secretion, ASC-deficient macrophages were fully defective in LeTx-induced caspase-1 autoproteolysis. This suggests that the absence of caspase-1 autoproteolysis—a parameter widely used to monitor inflammasome activation—alone is not sufficient to rule out inflammasome activation. In this regard, the general mechanisms of caspase-1 activation in inflammasome complexes may much resemble those governing activation of the apoptotic initiator caspases 8 and -9 in the death-inducing signalling complexes and the apoptosome, respectively [32] , [33] . We therefore propose a model in which NLRP1b directly recruits caspase-1 via homotypic CARD–CARD interactions to assemble a functional inflammasome complex in the cytosol of LeTx-sensitive macrophages. Unprocessed, but enzymatically active caspase-1 in the NLRP1b inflammasome triggers cytokine production and pyroptotic cell death. ASC-mediated clustering of multiple NLRP1b inflammasomes in specks further increases the local concentration of active caspase-1 dimers, promoting their proximity-induced autoproteolysis. While this may generally serve to stabilize the active protease, further analysis is required to understand why ASC specifically enhanced IL-1β secretion, but not cell lysis of macrophages exposed to low LeTx concentrations. Notably, caspase-1 activation in the NLRP1b inflammasome was associated with its ubiquitination, which occurred independently of ASC expression and caspase-1 autoproteolysis. Interestingly, caspase-1 ubiquitination was not limited to the NLRP1b inflammasome as it was also observed upon activation of the NLRP3, AIM2 and NLRC4 inflammasomes. Caspase-1 ubiquitination likely occurs downstream of caspase-1 activation in inflammasomes because the caspase-1 inhibitor Ac-YVAD-cmk prevented LeTx-induced caspase-1 post-translational modification. We therefore hypothesized that caspase-1 ubiquitination may represent a negative feedback mechanism that dampens inflammasome activation by targeting active caspase-1 for degradation by the proteasome. However, the proteasome inhibitor MG132 inhibited LeTx-induced pyroptosis and caspase-1 autoproteolysis altogether (data not shown), thus hampering investigation of the potential role of the proteasome in degrading inflammasome-activated caspase-1. However, future identification of the molecular machinery driving caspase-1 ubiquitination may shed light on its putative role(s) in inflammasome signalling. Regardless, we showed that the differential requirement of ASC for caspase-1 autoproteolysis and its biological effects also applies to mice challenged in vivo with LeTx. As in macrophages, LeTx-induced caspase-1 autoproteolysis in the spleen required ASC and a functional NLRP1b allele. Nevertheless, LeTx-challenged ASC-deficient mice released HMGB1—an endogenous danger signal released from pyroptotic cells—in circulation, suggesting normal cell death induction in vivo . Moreover, their serum contained significant amounts of IL-1β and IL-18, although the levels were detectably lower than in littermates expressing ASC. In contrast, mice lacking a functional NLRP1b allele were fully defective in both HMGB1 release and secretion of IL-1β and IL-18. As a result, ASC deletion failed to protect against LeTx-induced mortality, whereas the absence of a functional NLRP1b allele significantly delayed lethality. In conclusion, we showed that ASC is critical for LeTx-induced caspase-1 autoproteolysis and speck formation, but that these events are dispensable for NLRP1b inflammasome-mediated caspase-1 activation, cytokine secretion and cell death induction in susceptible macrophages and in toxin-intoxicated mice. Mice B6 Nlrp1b+ ASC −/− and B6 Nlrp1b+ Casp1 −/− mice and littermate controls used in this study were obtained by breeding B6 Nlrp1b+ (ref. 8 ) to Asc −/− (ref. 18 ) and Casp1 −/− (ref. 34 ) mice in a C57BL/6 genetic background, respectively. Asc −/− and Casp1 −/− mice were also backcrossed to a BALB/c genetic background for 10 generations. C57BL/6J, 129SVEV57 and BALB/c mice were originally purchased from Charles River and bred in-house. Animals were housed in individually ventilated cages under specific pathogen-free conditions, and studies were conducted under protocols approved by Ghent University and St Jude Committees on Use and Care of Animals. Macrophage differentiation and stimulation BMDMs were generated by culturing mouse bone marrow cells in L-cell-conditioned IMDM supplemented with 10% FBS, 1% non-essential amino acid and 1% penicillin–streptomycin for 6 days. BMDMs were seeded in 12-well plates, and the next day either left untreated or stimulated with LPS (5 μg ml −1 ) for 3 h prior to treatment with different concentrations of anthrax PA, and wild-type or proteolytically inactive LF (Quadratech). In some experiments, BMDMs were pretreated with the caspase-1 inhibitor Ac-YVAD-cmk (50 μM; Enzo Life Sciences) for 30 min prior to LeTx incubation. Alternatively, macrophages were primed with LPS for 3 h and then stimulated with 20 μM nigericin for 1 h or 5 mM ATP for 30 min. In other experiments, BMDMs were infected with S. typhimurium at m.o.i. of 10, 5 or 1 for 3 h in a CO 2 incubator at 37 °C, the last hour of which in the presence of gentamycin (50 μg ml −1 ). Alternatively, BMDMs were infected with F. tularensis at m.o.i. 30 for 3 h, the last hour of which in the presence of gentamycin (50 μg ml −1 ). Finally, cytosolic dsDNA delivery was performed by transfecting cells for 24 h with Lipofectamine-2000 reagent (Life Technologies) according to the manufacturer’s instructions. Western blotting Cell lysates, serum samples and spleen homogenates denatured in loading buffer containing SDS and 100 mM DTT were boiled for 10 min before SDS–PAGE-separated proteins were transferred to PVDF membranes. Immunoblotting with primary antibodies against caspase-1 (1/3,000, kind gift of Dr Peter Vandenabeele, Ghent University), ASC (1/1,000, AG-25B-0006, Adipogen), IL-1β (1/2,000, GTX74034, GeneTex), caspase-11 (1/1,000, NB120-10454, Novus Biologicals), Ub-HRP (1/1,000, sc-8017, Santa Cruz), HMGB1 (1/100, 18256, Abcam), and β-actin (1/20,000, NB600-501H, Novus Biologicals) was followed by secondary anti-rabbit and anti-rat HRP antibodies (1/5,000, 111-035-144 and 112-035-143, Jackson Immunoresearch). Ponceau S Solution was purchased from Sigma-Aldrich. Fluorescence and confocal microscopy B6, B6 Nlrp1b+ and B6 Nlrp1b+ ASC −/− macrophages grown on coverslips were either left untreated (mock) or stimulated with LeTx for 30 min after which the active caspase-1 FAM-YVAD-cmk FLICA probe (Gentaur Molecular Products) was added for another 45 min. Cells were fixed and mounted on glass slides using ProLong Gold Antifade reagent containing DAPI (Life Technologies). Fluorescence micrographs were taken on an Olympus microscope using a × 20 objective lens. Quantification of specks was performed in three micrographs and the mean grey value was determined in 10 cells using ImageJ software. Alternatively, cells grown on coverslips were treated with LeTx for 60 min, fixed in 4% paraformaldehyde and then stained with antibodies against ASC (1/400, AG-25B-0006, Adipogen) and caspase-1 (1/200, AG-20B-0042-C100, Adipogen). Secundary antibodies anti-mouse Alexa Fluor 488 and anti-rabbit Alexa Fluor 594 (1/250, A-11029 and A-11037, Invitrogen) were used. Slides were mounted in ProLong Gold Antifade reagent with Dapi (P36935, Invitrogen). Confocal micrographs were taken on an Olympus microscope using a × 60 objective lens. Quantification of specks was performed on 10 micrographs. Immunoprecipitation Treated BMDMs (12 × 10 6 cells per 10 cm dish) were lysed in 500 μl Cell Lysis buffer (10 mM Tris–HCl, pH 8, 0.15 M NaCl, 2% SDS) supplemented with 100 mM N -ethylmaleimide (Sigma) and a Complete Protease Inhibitor Cocktail tablet (Roche Applied science) and supernatants were collected. Lysates and supernatants were boiled for 10 min followed by sonication for 5 min. After centrifugation, supernatants and lysates were pooled and incubated with caspase-1-specific nanobody clone R2S40 that was developed in-house (1/100, VIB Nanobody Service Facility) on a rotating platform at 4 °C for 1 h. Subsequently, HA-beads were added and incubated overnight on a rotating platform at 4 °C. The next day, beads were washed three times before being resuspended in 1 × Laemmli buffer and boiled for 10 min. Eluted samples were analysed by SDS–PAGE. In vivo LeTx challenge Cohorts of 8–12 week-old male and female B6, B6 Nlrp1b+ and B6 Nlrp1b+ ASC −/− littermates were injected intraperitoneally with 100 μg PA+100 μg LF for 3 h before serum was collected for cytokine analysis, and spleen homogenates were prepared for immunoblotting. In other experiments, groups of B6, B6 Nlrp1b+ and B6 Nlrp1b+ ASC −/− mice were injected intraperitoneally with 200 μg PA+200 μg LF to monitor survival. Cytokine analysis Cytokine levels in cell culture medium and serum were determined by multiplex ELISA (Bio-Rad), IL1β ELISA (R&D Systems) and IL-18 ELISA (MBL international), according to the manufacturers’ instructions. LDH measurement Cell death levels were determined by LDH assay in culture medium according to the manufacturer’s instructions (Promega). RT–qPCR Total RNA was isolated using the Qiashredder and RNeasy Mini kits (Qiagen), according to the manufacturer’s instructions. RNA (1 μg) was used for cDNA synthesis with iScript reagents (Bio-Rad). Quantitative PCR on duplicate samples was performed using the LightCycler 480 SYBR Green master mix (Roche) and normalized to the housekeeping gene β-actin. Primers used were 5′-CAACAAGACTTGAACACAACGAG-3′ and 5′-CTCTCAATGACTGTGCTGGGTA-3′ for NLRP1b [8] ; and 5′-GTCGACAACGGCTCCGGC-3′ and 5′-GGTGTGGTGCCAGATTTTCT-3′ for β-actin. Statistics GraphPad Prism 5.0 software was used for data analysis. Data are represented with s.d. or s.e.m., as indicated. Statistical significance was determined by Student’s t -test for cell death and cytokine assays, and Kaplan–Meier analysis was used to analyse mortality; P <0.05 was considered statistically significant. How to cite this article: Van Opdenbosch, N. et al . Activation of the NLRP1b inflammasome independently of ASC-mediated caspase-1 autoproteolysis and speck formation. Nat. Commun. 5:3209 doi: 10.1038/ncomms4209 (2014).